Reply to: Testing the adaptive hypothesis of lagging-strand encoding in bacterial genomes 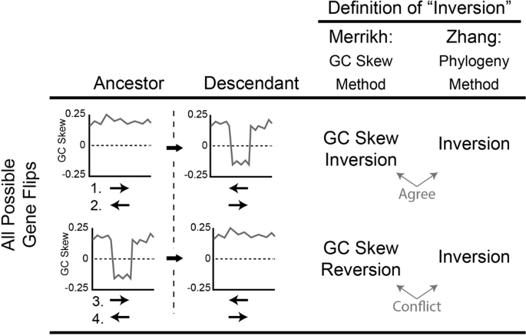Fig. 1: Comparison of gene “inversion” definitions and detection methods. The two studies use different definitions of “gene inversion”. For clarity, we use “Gene Flip” to mean any change-of-orientation event. Gene flips have two subtypes resulting in a gene having a negative GC Skew (upper graphs) or a positive GC skew (lower graphs). The Merrikh and Zhang definitions agree in the first scenario (upper graphs), but conflict in the second (lower graphs). As both gene orientation and GC skew sign (±) are important considerations, there are four possible circumstances (numbered 1–4) indicated under the GC skew plots. In case 1, a natively leading strand gene (indicated by the positive GC skew) undergoes a flip resulting in a GC skew inversion. In 2, a natively lagging-strand gene undergoes a flip, also resulting in a GC skew inversion. In 3, a leading strand gene with a negative GC skew flips, resulting in a GC skew reversion. In 4, a lagging-strand gene with a negative GC skew flips, resulting a GC skew reversion. Inference of positive selection We first compiled the nucleotide sequence alignment files produced by TimeZone v.1 and published in Ref. [4] . Alignments for genes determined to have a dN/dS value greater than 1 were input into PAML’s CodeML application. Likeliood ratio tests of models M1a (null hypothesis) versus M2a (positive selection) were used to determine if each gene is likely under positive selection at the 95% significance level. CodeML settings were based on established standards [19] . The fraction of all leading or all lagging-strand genes inferred to be under positive selection, and also having a dN/dS ratio >1 were calculated. Only genes fulfilling both criteria were considered to be under positive selection in our analysis. Fisher’s exact test was used to determine if the observed frequencies are significantly different for leading versus lagging-strand genes. GC skew calculation method comparison The GC Skew, defined as (G − C)/(G + C), was calculated for the leading strand sequence of whole-gene regions or using only nucleotides corresponding to the 1st, 2nd, or 3rd codon positions. Python scripts are publicly available at https://github.com/The1stMartian/GCskewAnalyzer . The Pearson Correlation coefficient was calculated for the whole-gene average method versus the indicated codon position-specific method (Supplementary Data 4 ). Independent phylogeny-based analysis vs. GC skew analysis Data are presented in Supplementary Data 5 . The program OrthoFinder 1.0 was used to identify all single copy orthologs between B. subtilis strain 168 and B. licheniformis strain ATCC 14580 using default settings. Gene orientations were annotated in Microsoft Excel based upon the replication origins and termini listed on the DoriC database [5] , [20] . 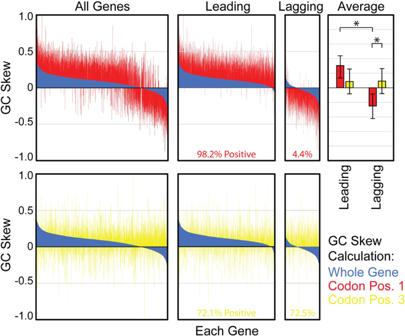Fig. 2: GC Skew values for whole-gene regions. Upper graphs: GC skew values are calculated using whole-gene regions (blue) or only codon position 1 nucleotides (red) for allB. subtilisgenes, leading strand genes only (Leading), or lagging-strand genes only (Lagging). Genes are sorted based upon the whole-gene GC skew resulting in the appearance of a curve. CP1 and CP3-based values are not independently sorted, allowing for direct comparison between data sets. The average GC skew values (Average) demonstrate that CP1-based GC skew values (red) are significantly different for leading versus lagging-strand genes, whereas CP3-based values (gold) are not. Additionally, CP1-based GC skew values are significantly different from CP3-based values for lagging-strand genes. Error bars represent the standard error of the mean. Significance was determined by the z-test, asterisk symbol (*) indicatesp= 0.0. The percentage of positive CP1-based GC skew values is shown at the bottom of the Leading and Lagging-strand gene graphs. Lower graphs: Whole-gene (Blue, same data as upper graphs) versus CP3-based GC skew values are shown. 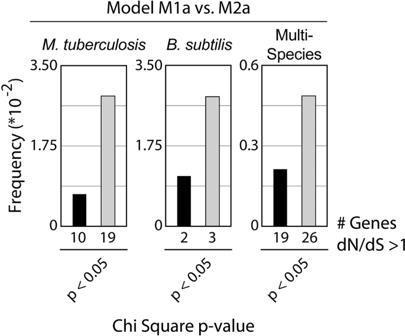Fig. 3: Lagging-strand genes are more frequently under positive selection. Likelihood ratio tests (LRTs) were used to compare site models M1a (neutral model) versus M2a (positive selection model) as a test for positive selection among genes with a dN/dS ratio >1. The frequency of genes better fitting the positive selection model at >95% significance are plotted (# genes under positive selection/total). Positive selection likely acts more frequently on lagging-strand genes inM. tuberculosis(Fisher’s exact testp= 0.049). An equivalent analysis is shown forB. subtilis(middle graph, Fisher’s exact testp= 0.12 for leading versus lagging-strand frequencies). Multi-species analysis: across species, genes under positive selection are more frequent in lagging-strand genes, confirming the results of our original analysis (right graph, Fisher’s exact testp= 0.005). Codon position-based GC skew values were calculated using custom Python scripts. Reporting summary Further information on research design is available in the Nature Research Reporting Summary linked to this article.